Distinct metabolomic signatures are associated with longevity in humans Alterations in metabolism influence lifespan in experimental models, but data in humans are lacking. Here we use liquid chromatography/mass spectrometry to quantify 217 plasma metabolites and examine their relation to longevity in a large cohort of men and women followed for up to 20 years. We find that, higher concentrations of the citric acid cycle intermediate, isocitrate, and the bile acid, taurocholate, are associated with lower odds of longevity, defined as attaining 80 years of age. Higher concentrations of isocitrate, but not taurocholate, are also associated with worse cardiovascular health at baseline, as well as risk of future cardiovascular disease and death. None of the metabolites identified are associated with cancer risk. Our findings suggest that some, but not all, metabolic pathways related to human longevity are linked to the risk of common causes of death. The mechanisms underlying a person’s ability to achieve longevity remain poorly understood. Much work has been done to identify the biological pathways that regulate lifespan in several model organisms including Caenorhabditis elegans ( C. elegans ), Drosophila and mice [1] , [2] . However, translating these findings to humans has been difficult. Identifying the mechanistic contributors to lifespan in humans is intrinsically challenging—largely due to the fact that numerous exposures, accumulating over the life course, can serve to modulate the influence of extant genetic determinants [3] , [4] . Despite this complex challenge, both the experimental literature and work to date in human studies point to alterations in metabolism as being the central and likely highest-yield targets for investigation [1] , [5] , [6] , [7] , [8] . This recognition has focused attention on the possibility that metabolomics technologies may shed light on pathways to longevity in humans [9] , [10] , [11] . By monitoring a large panel of purportedly related and unrelated small molecules in a given tissue (for example, circulating blood), metabolite profiling can provide ‘snapshot’ data reflecting the extent to which the biochemical pathways may be upregulated or downregulated in one individual compared with the next—thus integrating the influence of both endogenous and exogenous factors (that is, providing data on both genetic and environmental influences at a given point in time). Studies to date have analysed the cross-sectional associations of metabolites with clinical traits in aged adults [9] , [10] , [11] , [12] . By contrast, the extent to which distinct metabolite profiles captured earlier in life are prospectively associated with longevity in humans remains entirely unknown. Because the human metabolome is dynamic and constantly in flux, there have been concerns at the outset that detectable variation at a single point in time may not necessarily be associated with a clinical outcome years later. However, recent investigations in large cohorts have now demonstrated that alterations in circulating concentrations of distinct polar and lipid metabolites can predict the development of a specific disease phenotype, such as cardiovascular disease or diabetes or cancer, even a decade or more after the metabolite profile was originally captured [13] , [14] , [15] , [16] , [17] . These findings suggest that metabolite profiling could also help to uncover pathways related to overall survival and longevity. To this end, we performed a high-throughput metabolomics-based investigation in two well-phenotyped cohorts of middle-aged to older adults. We sought to identify circulating metabolite profiles associated with the future ability to achieve longevity, and assessed whether the metabolites identified were related to cardiovascular or cancer risk. We discovered polar compounds and lipid analytes related to longevity, including citric acid cycle intermediates and the bile acid taurocholate. Notably, only the citric acid cycle intermediates were concomitantly associated with cardiovascular risk and no longevity-related metabolites were associated with cancer risk, suggesting the possibility that some metabolic pathways to longevity in humans are distinct from those implicated in the development of common morbid diseases. Longevity outcomes We performed metabolite profiling on plasma samples collected from 2,327 participants of the Framingham Offspring Study who underwent a routine examination between 1991 and 1995. Of this ‘source’ study sample, a subset of 647 individuals had the chance to reach age 80 years by the end of the follow-up period on 31 December 2010 ( Supplementary Fig. 1 ). 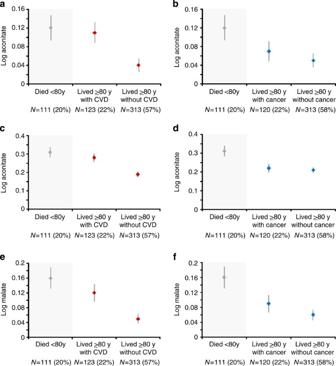Figure 1: Metabolites’ associations with longevity and morbidity profiles. Mean and s.e.m. values of selected log metabolite values are shown by morbidity profile in the first-stage study sample (N=647). Among individuals who lived to age⩾80 years, log aconitate (P=0.004), log-isocitrate (P=0.0005) and log malate (P=0.012) levels were significantly higher in those who ever developed cardiovascular disease compared with those who remained free of cardiovascular disease (a,c,e). These metabolites did not differentiate between individuals based on cancer morbidity (b,d,f). Comparisons were performed usingt-tests. Approximately half of the study participants were women ( Table 1 ). Of individuals with the chance to reach age 80 years, 79% ( N =514) succeeded in this regard. Of those who achieved longevity, 73% ( N =377) never developed cardiovascular disease and 25% ( N =126) developed cardiovascular disease after age 70 years ( Supplementary Table 1 ). Overall, 73% ( N =376) reached age ⩾ 80 free of cancer and 54% ( N =275) lived to age ⩾ 80 without ever developing either cardiovascular disease or cancer. Table 1 Sample characteristics. 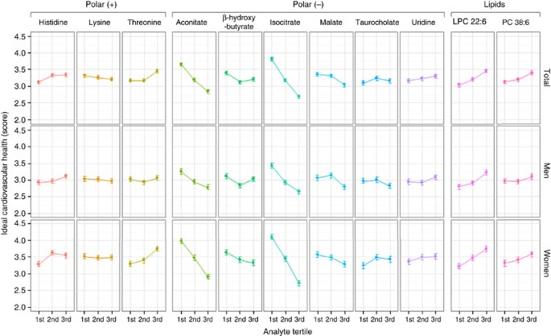Figure 2: Metabolite associations with ideal cardiovascular health. Mean and s.e. cardiovascular health scores are shown by tertile of selected analytes in the second-stage study sample (N=2,327) and by sex, where higher score denotes more ideal cardiovascular health. Analytes were selected based on their associations with longevity in the main study sample (N=647). Full size table Metabolite markers of longevity In the first stage of analyses, we performed age- and sex-adjusted logistic regression models in the sample with the chance to reach age 80 years ( N =647) and identified multiple distinct metabolites associated with longevity ( Table 2 and Supplementary Data 1 ). A Bonferroni-corrected P value threshold of 0.001 was used to account for multiple testing across the 37 clusters of intercorrelated metabolites (0.05/37; see Methods for additional details). In analyses additionally adjusting for previously reported correlates of attenuated lifespan, including smoking, the association of cotinine with longevity became non-significant, consistent with its generation as a by-product of nicotine. In these multivariable-adjusted models, isocitrate and taurocholate emerged as particularly significant correlates of longevity ( Table 2 ). Each s.d. increment in log-isocitrate was associated with a 37% lower odds of achieving longevity (adjusted odds ratio 0.63, 95% confidence interval (CI) 0.49–0.81; P =3.9E−04). Addition of isocitrate to a multivariable model comprised of traditional risk factors modestly, but significantly, improved the C -statistic from 0.72 to 0.74 ( P =0.0003). Similarly, each s.d. increase in log-taurocholate was associated with a 37% lower odds of achieving longevity (adjusted odds ratio 0.63, 95% CI 0.48–0.83; P =7.4E−04) and inclusion of taurocholate in the model improved the C -statistic from 0.72 to 0.75 ( P =0.0003). With respect to these associations, there was no significant effect modification by age or sex ( P >0.20 for all interaction terms). In addition to isocitrate, two other citric acid cycle intermediaries, aconitate and malate, were also associated with lower odds of achieving longevity ( P =0.002 and 0.001, respectively). Several other bile acids, including taurodeoxycholates ( P =0.002) and glycodeoxycholates ( P =0.007), also had nominal associations with longevity. The concordant associations of additional metabolites along these two metabolic pathways add further support to the primary findings. In secondary analyses performed using age thresholds of 85, 75 and 70 years to define longevity, results of the main analyses were similar ( Supplementary Tables 2–4 ). Table 2 Metabolites associated with attaining longevity defined as 80 years of age (first-stage sample: N =647). Full size table Metabolite markers of morbid disease and all-cause mortality In the second stage of analyses, we examined whether metabolites associated with longevity were also associated with all-cause mortality, cardiovascular risk and cancer risk in the full source sample ( N =2,327). In these analyses, a Bonferroni-corrected P threshold of 0.004 was used to account for multiple testing across the 12 metabolites found in association with longevity in the primary analyses (0.05/12). Over the total follow-up period of 16.7±3.6 years, there were a total of 439 deaths from all causes. 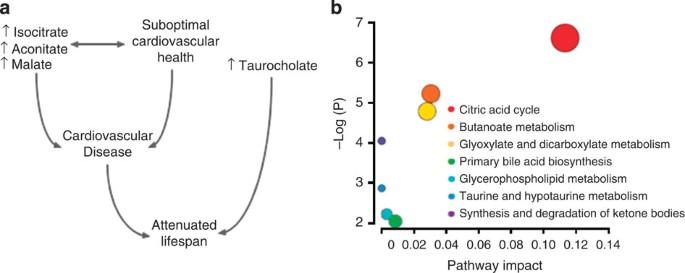Figure 3: Metabolite pathways observed in association with human longevity. Aggregate results of the current study suggest that higher circulating levels of certain citric acid cycle intermediates (isocitrate, aconitate and malate) are associated with shortened lifespan by increasing cardiovascular risk, whereas increased taurocholate is related to shorter lifespan independent of any concurrent associations with major morbid disease (a). Metabolomic pathway topology analysis highlights the potential importance of distinct pathways that comprise the human metabolome that are represented by metabolites associated with longevity in the current study (b). In multivariable analyses adjusting for age, sex, body mass index, systolic blood pressure, antihypertensive treatment, diabetes, smoking status and total/high-density lipoprotein cholesterol, we observed nominal to significant associations of aconitate ( P =0.0007), isocitrate ( P <0.0001), malate ( P =0.003) and taurocholate ( P =0.03) with the incidence of all-cause mortality ( Table 3 ). We observed a significant association of uridine with risk for all-cause mortality in the larger source sample, although the association of uridine with longevity did not meet the Bonferroni-corrected threshold of statistical significance in the subset longevity study sample ( Table 2 ). Table 3 Metabolites associated with all-cause mortality (second-stage sample: N =2,327). Full size table During the follow-up period, 358 of the total 2,327 individuals at risk developed a new-onset cardiovascular event (coronary heart disease, stroke or transient ischaemic attack or heart failure). Of the metabolites associated with longevity ( Table 2 ), only isocitrate was associated with incident cardiovascular disease ( Table 4 ). For each 1-s.d. increase in log-isocitrate, the risk of incident cardiovascular disease increased 22% ( P =0.002) in analyses adjusted for traditional cardiovascular risk factors. In multivariable-adjusted models, the citric acid cycle intermediate malate was similarly associated with greater cardiovascular risk ( P =0.009; Table 4 ) as well as decreased longevity ( Table 2 ). A total of 426 individuals developed a new diagnosis of cancer over the follow-up period. In multivariable analyses adjusting for age, sex, body mass index and smoking status, none of the metabolites listed in Table 2 were significantly associated with incident cancer (P ⩾ 0.06 for all, data not shown). Table 4 Metabolites associated with incident cardiovascular disease (second-stage sample: N =2,327). Full size table We sought to replicate findings from the second stage by performing analyses in the Malmö Diet and Cancer (MDC) cohort ( N =325) with the same metabolites (polar positive, polar negative and lipid compounds) assayed as in the Framingham cohort. We focused on the all-cause mortality, because the smaller sample size did not provide adequate power to examine individual categories of events. In the MDC replication sample ( Supplementary Table 4 ), there were a total of 36 deaths over a mean follow-up period of 15.8±2.4 years. In this smaller sample, and consistent with findings in the larger Framingham cohort, isocitrate was significantly associated with mortality in multivariable-adjusted models with a hazards ratio of 1.42 (95% CI 1.02–1.98; P =0.04). Malate demonstrated a similar multivariable-adjusted association with mortality (hazards ratio 1.37 (95% CI 0.99–1.91); P =0.059) whereas aconitate ( P =0.20) and taurocholate ( P =0.43) were not significantly associated with mortality. Metabolite markers of longevity and morbidity profiles We also investigated the association of metabolites with predefined morbidity profiles (survivors, delayers and escapers). Among individuals who lived to the age of 80 years, we compared the baseline values of select metabolites between those who developed cardiovascular disease or cancer and those who remained free of these disease conditions. Among individuals who achieved longevity, levels of the citric acid cycle intermediates were significantly different between those who developed cardiovascular disease compared with those who remained free of cardiovascular disease over the life course ( Fig. 1 ): log aconitate ( P =0.004), log-isocitrate ( P =0.0005) and log malate ( P =0.012). Baseline levels of these metabolites did not differentiate between individuals who achieved longevity with or without ever developing cancer ( Fig. 1 ; P >0.41 for all). Of the remaining metabolites identified in association with longevity in the main analyses ( Table 2 ), none significantly differentiated between morbidity profiles among individuals who lived to at least age 80 (data not shown). Figure 1: Metabolites’ associations with longevity and morbidity profiles. Mean and s.e.m. values of selected log metabolite values are shown by morbidity profile in the first-stage study sample ( N =647). Among individuals who lived to age ⩾ 80 years, log aconitate ( P =0.004), log-isocitrate ( P =0.0005) and log malate ( P =0.012) levels were significantly higher in those who ever developed cardiovascular disease compared with those who remained free of cardiovascular disease ( a , c , e ). These metabolites did not differentiate between individuals based on cancer morbidity ( b , d , f ). Comparisons were performed using t -tests. Full size image Metabolite markers of longevity and cardiovascular health To investigate the potential contribution of cardiovascular health to observed associations, we analysed the age- and sex-adjusted correlations of metabolites with the ideal cardiovascular health score at baseline in the source sample. The distribution of ideal cardiovascular health score and its components is shown in Supplementary Fig. 2 . Of the metabolites associated with longevity ( Table 2 ), those significantly related to the ideal cardiovascular health score at baseline included isocitrate as well as aconitate. Higher levels of these metabolites were associated not only with decreased longevity ( Table 2 ), but also worse cardiovascular health score: age- and sex-adjusted Spearman’s rank correlations were ρ= −0.29 ( P =6.6E−13) and ρ= −0.16 ( P =4.7E−05) for isocitrate and aconitate, respectively ( Fig. 2 and Supplementary Data 2 ). In addition, the lipophospholipid LPC 22:6 was associated not only with greater odds of longevity ( Table 2 ), but also with an increased ideal cardiovascular health score (Spearman rank correlation, 0.14; P =9.6E−09; Fig. 2 and Supplementary Data 2 ). Notably, the ideal cardiovascular health score at baseline accounted for a modest proportion of variation in these metabolites (<7%), as shown in Supplementary Table 6 . Associations between the full panel of metabolites and the ideal cardiovascular health score and its components are displayed in Supplementary Figs 3a–c . Figure 2: Metabolite associations with ideal cardiovascular health. Mean and s.e. cardiovascular health scores are shown by tertile of selected analytes in the second-stage study sample ( N =2,327) and by sex, where higher score denotes more ideal cardiovascular health. Analytes were selected based on their associations with longevity in the main study sample ( N =647). Full size image Pathway analyses Our overall results identified metabolites associated with longevity through potentially distinct pathways ( Fig. 3a ). Therefore, we used metabolomic pathway topology analysis to estimate the relative importance of metabolites associated with longevity and the pathways they represent (MetPA, Edmonton, Canada) [18] . On the basis of existing Homo sapiens data available from the KEGG database, results of these analyses are detailed in Supplementary Table 7 and highlight the potential relative importance of several distinct pathways ( Fig. 3b ). Figure 3: Metabolite pathways observed in association with human longevity. Aggregate results of the current study suggest that higher circulating levels of certain citric acid cycle intermediates (isocitrate, aconitate and malate) are associated with shortened lifespan by increasing cardiovascular risk, whereas increased taurocholate is related to shorter lifespan independent of any concurrent associations with major morbid disease ( a ). Metabolomic pathway topology analysis highlights the potential importance of distinct pathways that comprise the human metabolome that are represented by metabolites associated with longevity in the current study ( b ). Full size image Recent studies have sought to identify genetic as well as environmental factors that impact human lifespan [3] , [4] . Extending this prior work, we used high-throughput plasma metabolite profiling to identify ‘signatures’ of biochemical activity that may reflect the combined influence of endogenous and exogenous determinants—and offer a view of the potential pathways contributing to longevity among ambulatory adults living in the community. Using this approach, we identified metabolites not previously associated with lifespan in humans. Because cardiovascular diseases remain by far the leading cause of death worldwide [19] , maintenance of cardiovascular health over the life course would appear to strongly favour longevity [20] . Therefore, we also assessed the associations between plasma metabolites and the ability to maintain cardiovascular health. In our study, select citric acid cycle intermediates were associated with both worse cardiovascular health and decreased longevity. Although data in humans are scant, a substantial body of experimental data across several model systems has implicated citric acid cycle function in the regulation of lifespan in several model organisms. In yeast, citric acid cycle gene expression and activity are increased in the setting of increased longevity [21] , [22] . In Drosophila , the reduced gene expression of Indy (the plasma membrane transporter for citric acid cycle intermediates) extends lifespan [23] , [24] . Knocked down homologues of Indy have also been related to extended lifespan in C. elegans and dietary restriction phenotypes mice [25] , [26] , [27] . Furthermore, citric acid cycle genes are upregulated in long-lived Ames dwarf and Little mice [28] , and citric acid cycle function is preserved rather than reduced with aging in long-lived compared with short-lived strains of Brown–Norway rats [29] . Experimental studies have also reported on potential links between the specific citric acid cycle intermediates identified in our study (aconitate, isocitrate and malate) and longevity as well as cardiovascular phenotypes. Citrate is known to undergo stereospecific isomerization to isocitrate via cis-aconitate in the presence of aconitase; in turn, isocitrate undergoes oxidative decarboxylation in the presence of isocitrate dehydrogenase (IDH). Interestingly, the decreased expression of IDH has been shown to increase the generation of reactive oxidation species, DNA fragmentation, lipid peroxidation and concurrent mitochondrial damage [30] . Accordingly, in C. elegans , inactivation of IDH as well as aconitase genes via RNA interference has been shown to extend lifespan [31] . Addition of malate has also been reported to extend the lifespan in C. elegans while increasing the NAD to NADPH ratio [32] . In non-malignant cells, cytosolic IDH1 is known to be involved in lipid metabolism and glucose sensing, and mitochondrial IDH2 contributes to regulation of redox homeostasis [30] , [33] . Notably, mitochondrial IDH2 expression is particularly abundant in the heart [34] . In fact, experimental data have implicated mitochondrial IDH [35] , [36] , [37] as well as aconitase [35] , [38] and malate dehydrogenase [35] , [39] , in the development of cardiac hypertrophy. The extent to which the activity of these enzymes affects variation in the levels of peripherally circulating substrate metabolites is not yet known. In human malignant cells, mutations in the IDH1 and IDH2 isoforms appear to promote tumour survival [40] , [41] , [42] . Our data showed no association between isocitrate levels and cancer, though the extent to which circulating plasma levels relate to oncologic risk merits further investigation. Additional metabolites related to both better cardiovascular health and increased longevity included LPC 22:6. This docosahexaenoic acid-containing lipophospholipid has been related to increased fish intake [43] and decreased risk for developing diabetes [14] , but not previously associated with longevity. Our study also identified taurocholate as a marker of human longevity. For each 1-s.d. increase in log-taurocholate, the odds of achieving longevity decreased by almost 40%. Taurocholate is a bile acid conjugate of cholic acid and taurine, and experimental studies have suggested that taurine lowers risk for hypertension, stroke and other atherosclerotic diseases [44] . Interestingly, increased taurocholate was associated with reduced lifespan in the absence of any relation to risk for cardiovascular disease or for cancer. This finding suggests that certain bile acids may represent a pathway to longevity unrelated to cardiovascular or cancer risk per se . Bile acids are now recognized as signalling molecules that regulate not only cholesterol homeostasis but also glucose and energy metabolism [45] , [46] . Bile acids have been shown to induce energy expenditure, decrease body weight and enhance glucose tolerance by activating TGR5, a G protein-coupled receptor expressed in brown fat and muscle tissue [47] , [48] . In addition, intestinal infusion of taurocholate in an animal model was observed to substantially increase activation of the Akt signalling pathway [49] , a reported determinant of cellular senescence [50] , [51] . Because bile acids are actively involved in regulating their own synthesis through enterohepatic circulation, the degree to which higher or lower circulating plasma levels of taurocholate reflect overall bile acid activity is not well understood. Further research is needed to better understand relationship between taurocholate metabolism and human longevity. Several limitations of the present study merit consideration. Given the age range of our study cohort at baseline, few individuals in our study had the chance to live to age 90 or 100 years, which are definitions of human longevity that have been studied previously. Therefore, we considered longevity as living to age 80, and inclusion in our longevity study sample (as derived from the larger source sample) was dependent on a minimum age requirement at the baseline examination. However, the metabolites identified in the current study are distinct from those previously associated with older age [52] , and all reported associations in our study were significant in analyses adjusting for age as well as sex. Cause of death could not be precisely adjudicated in our study because detailed clinical information around the time of death was not available for all participants. It is important to note that our liquid chromatography–mass spectrometry (LC–MS) platform identifies a large number of metabolites that have not been assayed in other large study samples with similarly long-lived individuals, precluding the ability for complete validation of our main findings in a separate cohort. Thus, our findings should be considered hypothesis generating, while providing interesting results that are consistent with data from experimental literature. Because our study samples included only adults of European ancestry, the generalizability of our findings to individuals with broader demographic representation is unknown. Further investigations of metabolomic traits in more diverse cohorts with longitudinal follow-up data on adequately aged individuals appear warranted. Although we observed concordance in directionality of metabolite associations in both the primary FHS sample and the smaller-sized MDC replication sample, future studies in larger cohorts are also needed to further investigate possible additional metabolite associations with longevity that our samples were not adequately powered to detect. In summary, several polar compounds and lipid analytes were associated with longevity in our large, community-based cohort. The citric acid cycle intermediate, isocitrate, and the bile acid, taurocholate, demonstrated particularly significant associations with longevity. Lower circulating levels of isocitrate and other citric acid cycle intermediates were not only associated with longevity but were also associated with ideal cardiovascular health at baseline, with lower risk for developing cardiovascular events over the follow-up period and with greater likelihood of achieving longevity free of any cardiovascular disease. These findings suggest that alterations in the citric acid cycle activity are related to longevity at least partly through increasing risk for cardiovascular disease. In contrast, taurocholate demonstrated a significant association with longevity in the absence of any relations to either cardiovascular or cancer risk. Thus, our data indicate that some but not all metabolic pathways related to human longevity are linked to the risk of common causes of death. Study samples In 1971, the Framingham Offspring Study enrolled 5,124 individuals in a prospective community-based cohort study, as described previously [53] . All study participants have been followed longitudinally with quadrennial examinations. Plasma samples from a total of 2,526 participants, from the fifth examination (1991–1995), were analysed by metabolite profiling. After excluding 90 individuals with prevalent cardiovascular disease and 109 with missing clinical covariates, a total of 2,327 participants had complete information available, based on data collected from a physician-administered medical history, physical examination and routine laboratory tests. These individuals comprised the ‘source’ study sample. Of this source sample, 647 participants attended their fifth examination on a date that allowed the possibility of reaching age 80 years by the end of the follow-up period (31 December 2010). These individuals comprised the study sample for the first metabolite-discovery stage. All participants provided written informed consent. All study protocols were approved by the Boston University Medical Center Institutional Review Board. Selected findings from Framingham were examined for replication in the cardiovascular cohort of the MDC study, an investigation of 6,103 individuals originally enrolled between 1991 and 1996 as part of a longitudinal population-based epidemiologic cohort. All participants attending the first study visit underwent a standardized physical examination and medical history and routine laboratory tests. A total of 791 participants provided fasting plasma specimens that underwent metabolite profiling using at least one of the three main profiling methods described herein (for identifying polar positive, polar negative or lipid compounds) [54] . Of this sample, after excluding individuals with a history of cardiovascular disease or missing covariate data, plasma specimens from a total of 325 individuals were identified as having underwent metabolite profiling using all three of the exact same profiling methods as used in the Framingham analyses; these individuals were originally selected from the larger MDC study as part of a previously reported diabetes case-control study [13] . All study protocols were approved by the Institutional Review Board of Lund University, Sweden. All participants provided written informed consent. Assessment of longevity and related outcomes For the first stage of analyses in Framingham, we defined longevity as achieving age ⩾ 80 years during the follow-up period. We selected age 80 years as the prespecified threshold for longevity to maximize the total number of participants available for analyses given the baseline age and life expectancy in our cohort ( Supplementary Table 8 ). Thus, the primary longevity analyses were restricted to the individuals who had the ability to reach 80 years old during the follow-up period, as determined by their age at baseline and the length of follow-up. To further assess potential contributors to longevity, we categorized the individuals who achieved longevity as ‘survivors’ (developed either of the two major morbidities, cardiovascular disease or cancer, before age 70), ‘delayers’ (developed cardiovascular disease or cancer after age 70) and ‘escapers’ (never developed cardiovascular disease or cancer). All study participants were under longitudinal surveillance for the incidence of cardiovascular disease, cancer and death; all events were adjudicated by a panel of three investigators based on a review of medical records [55] . Incident cardiovascular disease was defined as new-onset coronary heart disease, heart failure or stroke. Information on cancer outcomes was collected from the medical history at routine Framingham examinations, and all reports of cancer were verified by a review of medical records including submitted pathology, surgery and autopsy reports [56] . Incident cancer was defined as a new diagnosis of malignant neoplasm, not including non-melanoma skin cancer [57] . Cause of death was determined based on review of medical records, death certificates and interviews with next of kin. Assessment of cardiovascular health We further assessed the role of cardiovascular comorbities in the longevity experience by constructing a cardiovascular health score based on the seven metrics identified by the American Heart Association (AHA) as ideal goals for risk reduction in the general population [58] . These parameters of ‘ideal’ cardiovascular health have been associated, in aggregate, with lower risk for both cardiovascular death and all-cause mortality [20] . Therefore, we calculated the ideal cardiovascular health score based on the following AHA criteria—untreated total cholesterol <200 mg dl −1 , untreated blood pressure <120/80 mm Hg, non-smoker within the prior 12 months, untreated fasting blood glucose <100 mg dl −1 , body mass index <25 kg m −2 , meeting ⩾ 2 of the AHA diet goals based on data collected from a validated food frequency questionnaire [59] and optimal physical activity defined as being in the upper quartile of the physical activity index [60] . Ideal diet was defined as meeting ⩾ 2 dietary goals given the very low frequency of individuals meeting ⩾ 4 dietary goals (2.1%); similar observations have been made in the NHANES cohorts [20] . The assessment of ideal diet involves assigning one point for each of the following [58] : daily intake of ⩾ 4.5 cups of fruits and vegetables; at least twice weekly intake of 3.5-ounce serving of fish; at least thrice daily 1-ounce services of fibre-rich whole grains; <1,500 mg daily of sodium; and no more than 36 ounces weekly of sugar sweet beverages. For data regarding fruit and vegetables intake that was not reported in cup units in the Framingham food frequency questionnaire, conversions were performed based on the USDA guidelines [61] . Data regarding whole-grain intake was converted from servings to ounces, based on recommendations of the US Whole Grains Council [62] . For estimating sugar sweet beverage intake, one can of soda was considered equivalent to 12 ounces. It should be noted that because the questionnaire did not capture data on added salt, assessment of salt intake was derived exclusively from the food and beverage survey. Because leisure-time physical activity duration was not assessed, we used the physical activity index assessment, which is known to be correlated with metabolic equivalent tasks [63] . Presence of any of these variables was assigned 1 point as part of a clinical score ranging from 0 to 7. Metabolite profiling Metabolite profiling was performed on plasma samples that were collected from study participants following an overnight fast and then stored at −80 °C before the metabolite profiling assays. Plasma metabolites were analysed using LC–MS. Metabolites were extracted using organic solvents (75% acetonitrile/25% methanol for positively charged polar compounds, 80% methanol for negatively charged polar compounds and isopropanol for lipids) before separation on an LC column. LC–MS data were acquired using either an AB SCIEX 4000 QTRAP triple quadrupole mass spectrometer (positively charged polar compounds and lipids) or an AB SCIEX 5500 QTRAP triple quadrupole mass spectrometer (negatively charged polar compounds). Polar, positively charged metabolites were separated using hydrophobic interaction liquid chromatography and analysed using multiple reaction monitoring in the positive ion mode [13] . Polar, negatively charged compounds, including central and polar phosphorylated metabolites, were separated using a Luna NH2 column (150 × 2 mm, Luna NH2, Phenomenex) and analysed using multiple reaction monitoring in the negative ion mode [64] . Lipids were separated on a Prosphere C4 HPLC column and underwent full scan MS analysis in the positive ion mode [14] . Collectively, >200 endogenous metabolites were reproducibly measured for comparative analyses. MultiQuant software (Version 1.2, AB SCIEX) was used for automated peak integration and manual review of data quality before statistical analysis [14] . We prepared calibration curves for each analytical queue using internal reference standards (including isotope-labeled leucine-13C, 15 N, isoleucine-13C6, 15 N, alanine-13C, glutamic acid-13C5, 15 N, taurine-13C2, trimethylamine-N-oxide-d9, and valine-d8 and the non-mammalian lipid 1-dodecanoyl-2-tridecanoyl-sn-glycero-3-phosphocholine), as previously described [13] , [14] , [65] . For all three profiling platforms, a pooled plasma sample was also run following every 20 samples, and the peak areas in samples were normalized to metabolite peak areas in the nearest pooled plasma. Statistical analysis All metabolite variables were natural log transformed due to skewed distributions. In the first stage study sample ( N =647), we used age- and sex-adjusted logistic regression models to examine the associations of metabolites with longevity. We then repeated logistic regression analyses with additional adjustment for body mass index, systolic blood pressure, antihypertensive treatment, diabetes, smoking status, total cholesterol, high-density lipoprotein cholesterol and log triglycerides. We used logistic regression analyses to examine the associations with the ability to achieve longevity given the age range of participants at baseline, precluding a time to event analysis. In the second stage, we examined all individuals with metabolite profiling in Framingham ( N =2327). For metabolites observed to demonstrate significant associations with longevity, we performed Cox proportional hazards models to analyse their associations with incidence of all-cause mortality, cardiovascular disease and cancer. Covariates included in all multivariable-adjusted models were selected based on reported associations with longevity phenotypes in community-based studies [66] , [67] , [68] . We also calculated Spearman rank correlation coefficients to assess the relation of each metabolite with the cardiovascular health score, with adjustment for age and sex. To account for multiple testing, we used a Bonferroni-corrected P value threshold for the primary analyses of longevity as the main outcome. The majority of metabolites studied are known to be correlated within biological groups (for example, amino acids, bile acids, urea cycle metabolites, lipids). Therefore, for each profiling method (polar positive, polar negative and lipid), we performed three separate cluster analyses to identify groups of closely correlated metabolites in the total sample of individuals who attended the fifth Framingham Offspring examination and had metabolite data available ( N =2,526). In this total sample, batch-adjusted residuals were generated for each metabolite (PROC MIXED) and these residuals were rank normalized using the Bloomberg method; we used cluster analysis (PROC VARCLUS) to classify correlated values into hierarchical groupings. Metabolite clusters were then formed based on principal components (using eigenvalue thresholds of 1). In total, we identified 37 clusters of intercorrelated metabolites, and these clusters were noted to contain metabolites associated with distinct biological pathways ( Supplementary Tables 9 to 11 ). Thus, based on previously described methods for accounting for multiple comparisons [69] , a P value threshold of 0.05/37=0.001 was selected for the primary statistical analyses of longevity as the outcome. To examine the extent to which analytes associated with longevity in the main analyses were also associated with outcomes related to longevity (that is, all-cause mortality, incident cardiovascular disease and cancer), we used a Bonferroni-corrected P value threshold of 0.004 (0.05/12) given the number of analytes ( N =12) found in association with longevity in the primary analyses. All analyses were performed using SAS, version 9.3 (SAS Institute, Cary, NC). Graphical displays were created using R v2.15.2 (R Development Core Team, Vienna, Austria). Accession codes: Data on the interaction between genotype and phenotype have been deposited in the database of Genotypes and Phenotypes (dbGaP) under accession codes pht002234.v3.p7, pht002566.v2.p7, pht002343.v2.p7, pht002567.v2.p7, pht002565.v2.p7 and pht002894.v1.p7. How to cite this article: Cheng, S. et al . Distinct metabolomic signatures are associated with longevity in humans. Nat. Commun. 6:6791 doi: 10.1038/ncomms7791 (2015).